Local determination of the amount of integration of an atom into a crystal surface Collective vibrational modes of crystal lattices, called phonons, determine fundamental material properties, such as their thermal and electrical conductivities. Bulk phonon spectra are influenced by point defects. More recently, the importance of phonons on nanostructures has come into the focus of attention. Here we show a spatially resolved phonon spectra of point defects that reveal distinctly different signatures for a cavity alone and an impurity atom fully integrated into the surface as opposed to one placed into a cavity. The spectra are indicative for delocalized phonons and localized vibrations, respectively, as confirmed by theory. Phonons of nanostructures are of current interest [1] , as phonons influence the electrical, optical, mechanical and thermal properties of materials [2] . Bulk phonon spectra, which were extensively investigated experimentally by spatially integrating methods [3] , are influenced by point defects [2] . Such an influence was demonstrated decades ago experimentally [4] by measuring the thermal conductivity and theoretically [5] by employing the Green’s function matrix method showing that bulk phonons scatter at lattice defects. It is by now well established that the two parts of the reflective index of refraction ñ determine two effects of defects onto phonon properties [6] . The real part of ñ is responsible for additional dispersion in the relationship between phonon frequency and wave vector. The lifetime of the phonons as described by the imaginary part of ñ decreases because of scattering effects. Today, the focus has shifted towards the influence of defects onto phonons for nanoscale objects as for example, thin diamond films [7] , single-walled carbon nanotubes [8] , [9] , [10] and semiconducting nanostructures [11] . In particular, the effect of structural defects on the low-temperature quantization of thermal conductivity was explored experimentally [12] and theoretically [9] . On the local scale, the inelastic electron tunnelling spectroscopy (IETS) signal of a d 2 I / dV 2 measurement by scanning tunnelling microscopy (STM) in the low-energy region contains information about phonon excitation on surfaces [13] . Different atomic distances within the so-called herringbone reconstruction of the Au(111) surface are reflected in the phonon spectrum [13] . Our method was recently used to study the electron–phonon interaction for Pb/Si(111) at the atomic scale [14] . Furthermore, phonons were utilized to identify the tip apex structure in a STM [15] and even its temperature [16] . High spatial resolution about the influence of point defects on surface phonon spectra was so far only provided by theory, for example, for phonons on pure metal surfaces and on surfaces with adatoms [17] , [18] . In this article, we explore local variations in phonon spectra induced by point defects via IETS and numerical simulations based on embedded atom method calculations. Our study shows that the smallest possible point defect, a missing substrate atom, induces a tiny increase in phonon density of states, which is nonetheless measurable by IETS. The replacement of a substrate adatom by another species leads to more pronounced change. The largest change is induced by a combination of the two. For the last case, however, the spectra take the form of an individual vibration. Our study thus shows that the smallest possible point defect, a missing substrate atom, shifts the phonon density towards lower energy. The replacement of a substrate adatom by another species leads to an overall increase in phonon density. For a combination of the two, the spectra take the form of localized vibrations. Such local-scale information was not accessible so far and gives unprecedented access into understanding the properties of material on the nanoscale. Surfaces We explore local variations in phonon spectra by investigating the influence of a Cu atom within a Ag(100) surface on the local phonon spectrum. For varying the degree of localization, we realize and investigate the scenarios depicted in Fig. 1a–c . A single Cu atom is either alloyed into the Ag(100) surface ( Fig. 1a ) or it is placed into a cavity that is larger than a single vacancy ( Fig. 1b ). In the latter case, the Cu atom might or might not touch the border of the cavity. Finally, we investigate a cavity without Cu in it ( Fig. 1c ). Details of the preparation of these structures and identification by STM are given in the Supplementary Figs 1–4 and the Methods section. A Cu atom alloyed into a cavity is imaged as a depression at most tunnelling parameters ( Fig. 1d ). A Cu atom placed into a cavity that is larger than one vacancy is imaged as a protrusion ( Fig. 1e ). The surrounding cavity is imaged as a depression. A single vacancy is imaged as a depression of larger apparent depth than the alloyed atom ( Fig. 1f ). 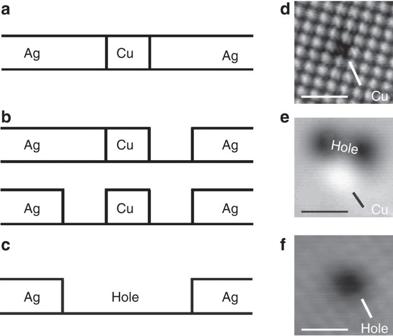Figure 1: Considered scenarios. (a–c) Schematic side view and (d–f) corresponding STM images, scale bar,: 1 nm: (a,d) Cu atom alloyed into the Ag(100) surface imaged as depression, 55 pA, 400 mV (b,e) Cu atom placed into a cavity of the Ag(100) surface, protrusions correspond to the Cu atom and depressions indicate the cavity in the Ag surface, which is imaged in grey, 1.1 nA, 302 mV (c,f) cavity in Ag(100) surface imaged as depression, 0.97 nA, 58 mV. Figure 1: Considered scenarios. ( a – c ) Schematic side view and ( d – f ) corresponding STM images, scale bar,: 1 nm: ( a , d ) Cu atom alloyed into the Ag(100) surface imaged as depression, 55 pA, 400 mV ( b , e ) Cu atom placed into a cavity of the Ag(100) surface, protrusions correspond to the Cu atom and depressions indicate the cavity in the Ag surface, which is imaged in grey, 1.1 nA, 302 mV ( c , f ) cavity in Ag(100) surface imaged as depression, 0.97 nA, 58 mV. Full size image Spectra of pristine surface To set the stage, we first discuss spectra recorded on the pristine Ag(100) before any additional surface treatment. These spectra show a point symmetric peak around the Fermi energy (V=0 mV) covering a range up to 30 mV with a peak at ~13 meV ( Fig. 2a ). Theory predicts the spectra to cover a smaller range ( Fig. 2b,c ). This difference in range is attributed to modulation and temperature broadening in the experimental case. In fact, the spectrum is slightly broader than the Au(111) spectrum presented before [13] as expected for the slightly larger phonon range. The shape of the experimental spectra is rather consistent with picking up the signal mainly from the surface layer ( Fig. 2b ) and less from the subsurface layer ( Fig. 2c ). Note that this signal has the same symmetry as phonon spectra recorded for Pd/Si(111) [14] and inverted symmetry to the spectra observed on Cu(111) and on Au(111) [13] . The reason for the latter inversion of symmetry has not yet been theoretically explored. Experimentally, we always observe the inverted symmetry on Cu(111) and Au(111), but only very rarely on Ag(100). For the qualitative discussion below, we will mainly compare our spectra with those calculated for the surface layer. 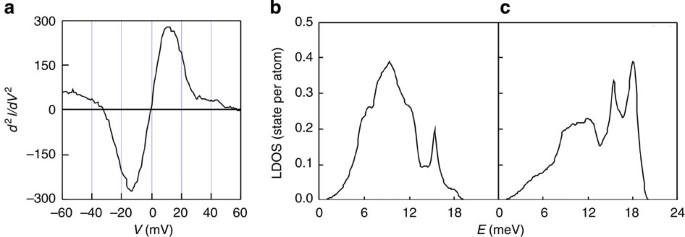Figure 2: Pristine Ag(100). (a) IET spectra on pristine surface,Vmod=10 mV,fmod=313.9 Hz (b,c) theoretical phonon LDOS for (b) surface layer (c) subsurface layer. Figure 2: Pristine Ag(100). ( a ) IET spectra on pristine surface, V mod =10 mV, f mod =313.9 Hz ( b , c ) theoretical phonon LDOS for ( b ) surface layer ( c ) subsurface layer. Full size image Spectra of alloyed atoms and holes The phonon spectra expected for the scenarios presented in Fig. 1a,b are shown in Fig. 3b–d . Our calculations predict that distinctly different signatures are expected. A single Cu adatom adsorbed on top of the surface leads to a distinct peak (at around 5 meV) ( Fig. 3a ), whereas alloying into the surface leads to a broad spectrum ( Fig. 3b ). The first one is indicative of a single vibrational level, whereas the latter represents a collective vibration. The same atom within a four-vacancy cavity ( Fig. 3c ) has a similar phonon spectrum as the atom alloyed into the surface, while being placed in a nine-vacancy cavity without any direct in-plane neighbours, the vibrational signature of the adatom is recovered ( Fig. 3d ). The phonon local-density-of-states (LDOS) from the Ag surface atoms differ only marginally for the different adsorption geometries ( Fig. 3a–d , orange line). Such slight variations will not be detectable in the experiment. We thus mainly concentrate on the spectra taken directly above a Cu atom, starting with the alloyed surface. 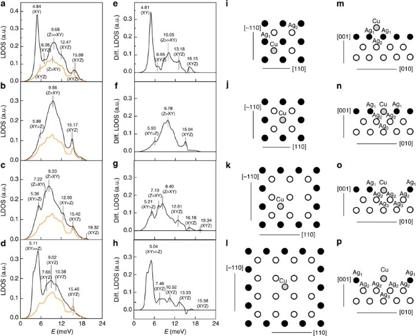Figure 3: Theoretical phonon spectra for four different scenarios. (a–d) Calculated phonon LDOS for the surface layer of Ag(100) with the Cu adatom (black line) and for the ideal Ag(100) (orange line) (e–h) difference LDOS between the Cu covered and ideal Ag(100) (i–p) schemes of calculated arrangements: (i–l): top view (m–p) side view: (a,e,i,m) Cu adatom situated on Ag(100), (b,f,j,n) Cu adatom integrated into single vacancy, that is, alloyed into the surface, (c,g,k,o) Cu adatom in cavity of four vacancies, (d,h,l,p) Cu adatom in cavity consisting of nine vacancies. Positions of maxima of vibrational modes are indicated in meV, and polarizations of these modes are shown. Figure 3: Theoretical phonon spectra for four different scenarios. ( a – d ) Calculated phonon LDOS for the surface layer of Ag(100) with the Cu adatom (black line) and for the ideal Ag(100) (orange line) ( e – h ) difference LDOS between the Cu covered and ideal Ag(100) ( i – p ) schemes of calculated arrangements: ( i – l ): top view ( m – p ) side view: ( a , e , i , m ) Cu adatom situated on Ag(100), ( b , f , j , n ) Cu adatom integrated into single vacancy, that is, alloyed into the surface, ( c , g , k , o ) Cu adatom in cavity of four vacancies, ( d , h , l , p ) Cu adatom in cavity consisting of nine vacancies. Positions of maxima of vibrational modes are indicated in meV, and polarizations of these modes are shown. Full size image The spectrum recorded at some distance from the alloyed Cu atoms and above the Cu atom has the same signature ( Fig. 4a ). However, intensity and position of the maxima differ. For elucidating this difference, we subtract the spectra from each other. This procedure is equivalent to subtracting the pristine surface spectrum with the advantage of eliminating possible tip effects. The point symmetric peak in the difference spectrum ( Fig. 4b , orange line) is clearly beyond the noise level. This is corroborated by a difference spectrum from the same series between two spectra recorded on the surface ( Fig. 4b , black line). As demonstrated in this example, changes in the spectra are tiny and, in the following, we directly present the relative signal with respect to the pristine surface. Keep in mind that the phonon signal is only ~2% of a typical IETS signal of molecular vibrations [13] , which already is only about 0.1% of the total tunnelling current [19] . 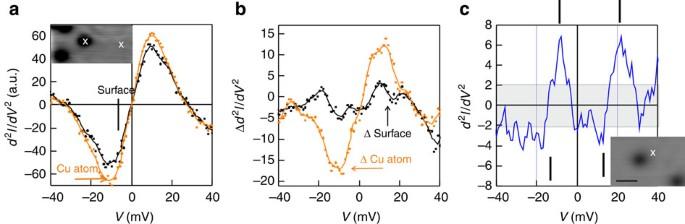Figure 4: Cu atoms integrated in crystal. IET spectra withVmod=10 mV,fmod=387.3 Hz: (a) spectra about 2 nm away from alloyed atoms (black line) and on alloyed atom (orange line) as indicated by crosses in inset (50 mV, 0.11 nA). (b) Difference spectra: in orange between spectra on Cu atom and on Ag surface, and in black between two spectra recorded on Ag surface (black). (c) Difference between IET Spectra at distance of 0.7 nm from centre of alloyed atom and on surface for the geometry shown in inset (50 mV, 0.1 nA, scale bar: 1 nm); grey shaded region indicates noise level. Figure 4: Cu atoms integrated in crystal. IET spectra with V mod =10 mV, f mod =387.3 Hz: ( a ) spectra about 2 nm away from alloyed atoms (black line) and on alloyed atom (orange line) as indicated by crosses in inset (50 mV, 0.11 nA). ( b ) Difference spectra: in orange between spectra on Cu atom and on Ag surface, and in black between two spectra recorded on Ag surface (black). ( c ) Difference between IET Spectra at distance of 0.7 nm from centre of alloyed atom and on surface for the geometry shown in inset (50 mV, 0.1 nA, scale bar: 1 nm); grey shaded region indicates noise level. Full size image Experimentally, the alloyed Cu atom exhibits a higher phonon density than the pristine substrate. Indeed, subtraction of the calculated LDOS on the ideal Ag(100) surface ( Fig. 3f ) shows that the LDOS is in all cases increased as compared with the ideal surface, as in the experiment. Also, the overall shape of the difference spectra in theory and experiment is similar. Furthermore, the experimental signal shows some spatial dependence. No deviations from the surface signal are observed beyond two atomic distances away from the defect. A tiny difference in signal between the spectra recorded at about one atomic distance (~0.3 nm) from the centre and a further atom away (~0.7 nm) is detectable ( Fig. 4c ). Thereby, the signal is reduced in the region up to ~15 mV, and it is increased up to ~30 mV as compared with the spectrum on the alloyed atom. In general, a change between signal reduction and increase is observed at (27±6) mV. This hints to a different spatial dependence of point defect-induced increases in phonon density in dependence of energy. For a visual impression of the spatial extend of this effect, see the Supplementary Fig. 5 and Supplementary Discussion . The spectra change more markedly for a Cu atom that is pushed into a sputter hole. Distinct peaks of much larger intensity (by one to two orders of magnitude) are observed at ~6 and ~28 mV ( Fig. 5b ). These cannot be attributed to phonon modes, that is, collective vibrations, because of the large intensity. For this Cu adatom within the non-perfect surface, that is, with less nearest neighbours, the two peaks might tentatively be attributed to the frustrated translations and the stretch mode vibration, respectively, of a single adatom on a surface, that is, the maxima in Fig. 5b result from vibrations of a single particle. A lower energy peak at around 5 meV is in surprising agreement with the one observed in theory. The additional peak at higher energy in the experiment might result from the difference in geometry, in particular the less symmetric arrangement. In summary, the qualitative features observed in the experiment are well reproduced: an alloyed atom is integrated into collective vibrations, while an adatom within a larger cavity retains the vibrational signature of an individual adsorbate. 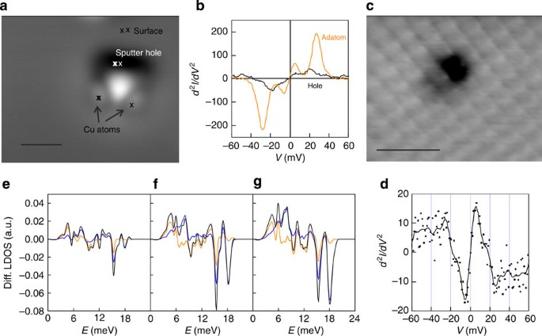Figure 5: Phonon spectra in sputter cavity. (a–d) STM images and IET spectra (a,b) for Cu atoms in sputter cavity (c,d) sputter cavity alone: (b) on cavity in black and on adatom in orange;Vmod=6 mV,fmod=378 Hz. (d) on cavity in (c);Vmod=6 mV,fmod=374.1 Hz; (a) 70 mV, 0.71 pA, scale bar, 1 nm (c) −5 mV, 77 nA; scale bar, 1 nm. (e–g) Calculated phonon LDOS for cavities of different size after subtraction of the ideal Ag(100) LDOS; surface layer (orange line), subsurface layer (blue line) and sum of both layers (black line) after a Gaussian broadening by 0.5 meV: (e) single vacancy (f) four vacancies (g) nine vacancies. Figure 5: Phonon spectra in sputter cavity. ( a – d ) STM images and IET spectra ( a , b ) for Cu atoms in sputter cavity ( c , d ) sputter cavity alone: ( b ) on cavity in black and on adatom in orange; V mod =6 mV, f mod =378 Hz. ( d ) on cavity in ( c ); V mod =6 mV, f mod =374.1 Hz; ( a ) 70 mV, 0.71 pA, scale bar, 1 nm ( c ) −5 mV, 77 nA; scale bar, 1 nm. ( e – g ) Calculated phonon LDOS for cavities of different size after subtraction of the ideal Ag(100) LDOS; surface layer (orange line), subsurface layer (blue line) and sum of both layers (black line) after a Gaussian broadening by 0.5 meV: ( e ) single vacancy ( f ) four vacancies ( g ) nine vacancies. Full size image Spectra of holes The signal strength above the Cu atom is too large to result from phonons. This point is corroborated by spectra recorded in the same measurement in the adjacent cavity ( Fig. 5b , black line). In contrast, intensity and shape of the spectra in the hole are indicative of phonons. In this particular case, the phonon density has maxima at ~5 meV and ~19 mV. Such values reoccur for cavities of different sizes, though often only one peak is observed. Note that the difference signal seems to get negative at larger energy. These general features are shown in better resolution for the small cavity shown in Fig. 5c . There is a prominent peak at ~6 meV, but the signal is negative above 19 meV ( Fig. 5d ). Thus, for holes the higher energy side of the surface phonon spectrum is reduced as compared with the pristine surface spectrum and the lower energy side is enhanced. This is equivalent to a downshift in the phonon density. This is in agreement with the calculated difference spectra. In Fig. 5e–g we show not only the spectrum expected for the topmost layer, but also for the subsurface layer, as we expect this to contribute in experiment, increasingly with increasing cavity size. The low energy positive peaks in Fig. 5e–g can be attributed to large horizontal vibrational displacements of the cavity edge atoms and to vertical displacements of the cavity bottom atoms. The high energy large negative peaks can be explained by occurrence at these energies of the pristine Ag(100) surface states mostly localized in the second atomic layer 27 and subtracted from the cavities LDOS. Including this second layer enhances the negative part of the spectrum. Though the fine details of the theoretical spectrum are not observable in experiment because of temperature and modulation broadening, the qualitative agreement is excellent. Theory further suggests that the relative cavity size might be determined from the phonon spectra in future as the intensity reduction in phonon spectra grows with cavity size. In conclusion, we show that IETS can be used to determine the amount of integration of an atom into a surface, information, which has not been available so far on the nanoscale. It can now be extended to other systems, to get a systematic picture about the influence of different substituents, differently integrated into the surface, on local phonon spectra. Understanding and control of defects is promising to tailor material properties that are influenced by phonons, in particular of surfaces and nanoscale material. Parts of surfaces might be manipulated for specific catalytic properties, which are likewise influenced by phonon properties by, for example, a change in adsorption and/or desorption probabilities. Tailored nanoparticles may in turn be investigated by IETS, if they are deposited on an inert surface, as done here. Surface preparation STM measurements are performed with a low-temperature STM under ultrahigh vacuum conditions [20] (base pressure <2 ·10 −10 mbar). The Ag(100) surface is cleaned by several cycles of sputtering with Ar + ions at p Ar =3 · 10 −5 mbar for 20 min and then annealing to 950 K for 3 min. After cleaning, the surface is further treated in two ways: first, for producing a dilute surface alloy, 0.003 ml to 0.13 ml of copper are deposited at room temperature with deposition rates between 0.001 ml min −1 and 0.01 ml min −1 (ref. 21 ). The substrate is held at room temperature for another 5 min before quenching the structures by cooling to ~50 K. The sample is then transferred into the STM, in which the measurements are performed in constant current mode at 5 K (ref. 21 ). An alloyed Cu atom is imaged at most tunnelling conditions as an apparent depression ( Fig. 1d ). Second, vacancy islands are produced by a mild sputter pulse (Ar + , 0.4 keV, I<0.01 μA, 3 s) with the surface at 100 K [22] , that is, below the onset of vacancy diffusion. At this temperature, the argon stays implanted in the surface. After the sputtering, the sample is directly cooled to ~50 K and transferred into the STM. The cavities created by sputtering are generally larger than one vacancy. Thus, lateral force manipulation is used to refill the cavity. A final vacancy is stable towards filling. Atomic resolution images are used to determine the size of the remaining cavity. Finally, we deposit Cu onto the sputtered surface. We again use lateral manipulation to transfer an individual Cu atom into a cavity. In contrast to the first preparation, this Cu atom has less nearest neighbours. It is imaged as a protrusion. Which of the different protrusions within a cavity corresponds to the Cu atom is known from the preceding manipulation series. Details of these procedures and the experimental identification of them are given in the supporting online material. After Cu deposition at room temperature, the larger Ag(100) terraces are covered by islands of monatomic height and quadratic shape with areas between 1 and 40 nm 2 ( Supplementary Fig. 1a ) [1] , whereas the smaller terraces look unchanged at first sight ( Supplementary Fig. 1b ). At enhanced contrast, depressions within the surface layer are observed ( Supplementary Fig. 1c ). The number of depressions is proportional to Cu coverage in the investigated range between 0.01 and 0.05 ml. Furthermore, they are only observed for deposition temperatures above 220 K. At regular tunnelling conditions, the depressions have an apparent depth of 6 pm ( Supplementary Fig. 1d,e ). In images of atomic resolution, each depression has the size of one atom only ( Supplementary Fig. 1f ). Moreover, the depressions turn into protrusions at some voltages ( Supplementary Fig. 1g ). Thus, each depression corresponds to one alloyed atom within the surface layer. Calculations suggest that alloying results from exchange diffusion on the terraces [2] (see inset of Supplementary Fig. 1h ). Indeed, the alloy density is independent from the distance to the step edge for distances > ~12 nm ( Supplementary Fig. 1h ). Some variations close to the step edge might result from a change in energy barrier of exchange diffusion at closer distance and/or from step fluctuations, but are not of importance here. The vacancies produced by a mild sputter pulse are shown in Supplementary Fig. 2 and resized as shown in Supplementary Fig. 3 . The same method is used to push a Cu atom into a vacancy ( Supplementary Fig. 4 ). Inelastic electron tunnelling spectroscopy In IETS, the second derivative of the tunnelling current with respect to the bias voltage ( d 2 / dV 2 ) is recorded in lock-in technique. Here, we superimpose the bias voltage with a sinusoidal modulation voltage of 5–15 mV (peak-to-peak) at a frequency of some hundred hertz. A point symmetric signal is indicative of an inelastic feature [19] . As recently corroborated by other groups [14] , [23] , we assign such a signal close to the Fermi energy to the phonons [13] . Some spectra displayed represent average spectra taken on equivalent sites. Some spectra a smoothed by averaging five adjacent points; the original data are shown as points. All features discussed were at least seen three times on similar objects. They do not differ within tip positioning precision (±0.05 nm), if measured repeatedly on the same object. Theory For understanding the experimental results, we calculate the local phonon density of states for the ideal surface and different arrangements that correspond to the ones explored experimentally. These consist of cavities containing one, four or nine vacancies, a single Cu adatom adsorbed on the surface and the same cavities incorporating one Cu adatom. We model the phonon spectrum of the Ag(100) surface using an embedded atom method [24] . Parameters of the method are determined by fitting to experimental data such as elastic constants, equilibrium lattice constants, sublimation energy and vacancy formation energy of pure Ag and Cu. The pair potential component Ag–Cu is constructed in the form proposed in ref. 25 . To obtain the equilibrium configuration at zero temperature, we relaxed the surface using the molecular dynamics technique based on the embedded atom method interaction potentials. A thin-film model of a two-dimensional periodic slab consisting of 31 atomic layers of Ag(100) is used to simulate a semi-infinite Ag metal. This thickness is sufficient to avoid interference effects related to opposite surfaces. We use (4 × 4) super cells for one vacancy, (5 × 5) ones for four vacancies and (6 × 6) ones for nine vacancies to exclude direct adatom–adatom or vacancy–vacancy interaction. The calculations of phonon spectra were carried out by the dynamical matrix method. The local vibration densities of states were obtained by projecting eigenmodes onto atoms of interest in a given ( x + y or z ) direction. As it is not possible to separate the different contributions in the experiments, average spectra over all polarizations DOS( x )+DOS( y )+DOS( z ) are displayed. However, we label the maxima with the corresponding polarization direction. How to cite this article: Volgmann, K. et al. Local determination of the amount of integration of an atom into a crystal surface. Nat. Commun. 5:5089 doi: 10.1038/ncomms6089 (2014).